NF-κB non-cell-autonomously regulates cancer stem cell populations in the basal-like breast cancer subtype Patients with triple-negative breast cancer display the highest rates of early relapse of all patients with breast cancer. The basal-like subtype, a subgroup of triple-negative breast cancer, exhibits high levels of constitutively active NF-κB signalling. Here we show that NF-κB activation, induced by inflammatory cytokines or by epigenetically dysregulated NIK expression, cell-autonomously upregulates JAG1 expression in non-cancer stem cells. This upregulation stimulates NOTCH signalling in cancer stem cells in trans , leading to an expansion of cancer stem cell populations. Among breast cancers, the NF-κB-dependent induction of JAG1 and the NOTCH-dependent expansion of the cancer stem cell population occur only in the basal-like subtype. Collectively, our results indicate that NF-κB has a non-cell-autonomous role in regulating cancer stem cell populations by forming intratumoural microenvironments composed of JAG1-expressing non-cancer stem cells with a basal-like subtype. Gene expression studies have established five breast cancer subtypes: luminal-like, v-erb-b2 avian erythroblastic leukemia viral oncogene homolog 2 (ERBB2)-enriched, basal-like, claudin-low and normal-breast-like [1] , [2] , [3] . The luminal-like subtype is characterized as displaying an oestrogen-receptor-positive (ER + ) and progesterone-receptor-positive (PR + ) phenotype, whereas the basal-like and claudin-low subtypes constitute the majority of triple-negative breast cancers (TNBCs; that is, ER − , PR − and ERBB2 − ). Although selective oestrogen-receptor modulators, aromatase inhibitors and trastuzumab are effective drugs for treating the luminal-like and ERBB2-enriched subtypes, TNBC displays high malignancy and exhibits a poor prognosis in response to various therapies [4] . To elucidate the signalling pathways that contribute to the malignant TNBC phenotype, we investigated NF-κB because NF-κB activation in TNBC is significantly higher than in other subtypes [5] . The NF-κB family consists of five members, namely, p50, p52, RelA, RelB and c-Rel, which form homo- and heterodimers to activate the transcription of target genes responsible for inflammation, immunoregulation and cell differentiation [6] . When forming complexes with members of the IκB family, including IκBα, IκBβ, IκBε, p105 (a precursor to p50) and p100 (a precursor to p52), NF-κB is transcriptionally inactivated due to its cytoplasmic sequestration. In the canonical pathway, many stimuli, including various cytokines and bacterial and viral products, induce the IκB kinase β (IKKβ)-catalysed phosphorylation of IκBα and its proteasomal degradation, which is followed by the nuclear translocation of p50-RelA heterodimers [7] . The non-canonical pathway is activated by receptors that are required for the formation of lymphoid organs and lymphocyte development, such as the lymphotoxin-β receptor, the receptor activator of NF-κB (RANK) and CD40. This pathway induces the IKKα-catalysed phosphorylation of the C-terminal half of p100, which sequesters RelB to the cytoplasm. This process leads to the polyubiquitination-dependent processing of p100 to p52, which is followed by the nuclear translocation of the p52-RelB heterodimers [8] . Most importantly, because of various negative regulators, activation of the two pathways is largely transient, enabling homoeostasis in inflammatory or immune responses [9] . Nevertheless, TNBC undergoes constitutive, strong NF-κB activation. Furthermore, the adenovirus-mediated expression of the non-degradable IκBα super-repressor (IκBαSR), in which Ser-32 and -36 (the residues phosphorylated by IKKβ) were substituted with alanine, blocked NF-κB activation and thereby inhibited the growth of several TNBC cell lines [5] . This result suggests that constitutive NF-κB activation has a critical role in TNBC malignancy. Cancer stem cells (CSCs), a subpopulation within a tumour, can self-renew and differentiate into various tumour cell types, thereby reconstituting intratumoural heterogeneity [10] . Moreover, CSCs are highly tumorigenic, relatively resistant to conventional chemotherapy and radiotherapy and involved in both tumour initiation and metastasis [11] . Therefore, the role of NF-κB activation in regulating CSC populations in TNBC is of particular interest. Although most previous studies have proposed that NF-κB activation in CSCs cell-autonomously regulates the CSC population, the molecular mechanisms by which NF-κB regulates CSCs are not fully understood [12] , [13] , [14] , [15] . Furthermore, because each breast cancer subtype is derived from mammary epithelial cells at a distinct differentiation stage, the molecular mechanisms for regulating CSC population are likely to differ among subtypes [16] , [17] , [18] , [19] . In this study, we sought to determine the role of NF-κB in regulating the CSC population in the basal-like breast cancer subtype and identified a subtype-specific, NF-κB-JAG1 axis that regulates CSC population size. NF-κB regulates CSC population in the basal-like subtype To analyse the relationship between NF-κB and the CSC population, we first assessed the correlation between NF-κB activation and the CSC population size, defined as the CD24 − CD44 high EpCAM + fraction [20] ( Fig. 1a ) or the ALDEFLOUR + fraction ( Fig. 1b ) (refs 21 , 22 ). Interestingly, the CSC population sizes in the basal-like cells were clearly correlated with the NF-κB activation levels in both CSC definitions ( Fig. 1a ). In contrast, a correlation between NF-κB activation and the size of the ALDEFLOUR + CSC fractions was scarcely observed in either the luminal-like or the claudin-low cells, although all of the claudin-low cell lines showed high-NF-κB activation levels ( Fig. 1b , the CD24 − CD44 high EpCAM + fractions were not recognized in the luminal-like and claudin-low subtypes, as shown in Fig. 1a ). These results led us to hypothesize that NF-κB may regulate CSC populations, specifically in basal-like cells. To confirm this hypothesis, we generated both ‘low-NF-κB cells’, in which IκBαSR was expressed to block NF-κB activation, and ‘high-NF-κB cells’, in which the constitutively active form of IKKβ (IKKβEE, generated by converting Ser-176 and Ser-180 in the activation loop into glutamic acid) or wild-type IKKβ was expressed to enhance NF-κB activation ( Fig. 1c ). The low-NF-κB cells showed a reduced CSC population, whereas the high-NF-κB cells showed an expanded CSC population in basal-like cells ( Fig. 1d , Supplementary Fig. S1 ). The modulation of NF-κB activation did not affect cell growth or survival ( Supplementary Fig. S2 ). However, this NF-κB-dependent regulation of the CSC population was not observed in the claudin-low or luminal-like cells ( Fig. 1e ). Under conditions in which approximately 90% of the mammospheres were derived from a single cell ( Supplementary Fig. S3 ), the low-NF-κB cells showed reduced mammosphere formation, whereas the high-NF-κB cells showed enhanced formation in basal-like cells ( Fig. 1g ). However, this NF-κB-dependent regulation of sphere-formation ability was not observed in the claudin-low or luminal-like cells ( Fig. 1h ). Tumour necrosis factor-α (TNFα) is a well-known cytokine that induces NF-κB activation and is involved in tumour malignancy [23] . TNFα stimulation, which induced RELB expression (indicating NF-κB activation), significantly expanded the CSC population ( Fig. 1i ) and enhanced the mammosphere-forming ability ( Fig. 1j ) of the basal-like cells. To further confirm the NF-κB-induced CSC population expansion, we analysed the effects of NF-κB activation on tumorigenicity. HCC1937 cells and cells containing modulated NF-κB activation were injected with Matrigel into the mammary fat pads of NOD/SCID mice, and palpable tumours were counted 10 weeks after injection. The low-NF-κB cells showed significantly lower tumorigenicity than the control cells, and the high-NF-κB cells displayed substantially higher tumorigenicity. 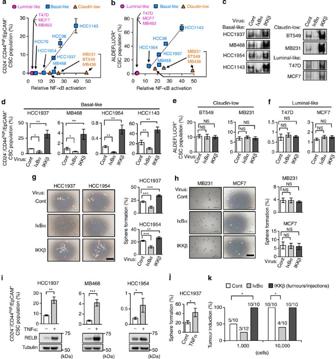Figure 1: NF-κB regulates the CSC population in basal-like breast cancer cell lines. (a) The correlation between constitutive NF-κB activation and the CD24−/CD44high/EpCAM+CSC population in various breast cancer cell lines. A linear regression analysis of values derived from the basal-like cell lines is shown as a dotted line (n=3, mean±s.d.,P=0.011; Pearson’s correlation coefficient). Relative NF-κB activities were determined as described in Methods. (b) The correlation between constitutive NF-κB activation and the ALDEFLUOR+CSC population in various breast cancer cell lines. A linear regression analysis of values derived from the basal-like cell lines is shown as a dotted line (n=3, mean±s.d.,P=0.015; Pearson’s correlation coefficient). (c) EMSA of NF-κB activation in control, IκBαSR and IKKβ-expressing breast cancer cells. (d) The percentages of the CD24−/CD44high/EpCAM+CSC populations (n=3, mean±s.d.; Student’st-test) in basal-like cell lines with various NF-κB activation levels. (e,f) The percentages of the ALDEFLUOR+CSC populations (n=3, mean±s.d.; Student’st-test) in the claudin-low (e) and luminal-like (f) cell lines with various levels of NF-κB activation. (g,h) NF-κB regulates the sphere-forming ability of basal-like cells (g), but not that of claudin-low and luminal-like cell lines (h); images showing sphere formation. Scale bar, 500 μm. (i) Fluorescence-activated cell sorting analysis of the CSC population in basal-like cell lines with or without TNFα treatment (10 ng ml−1) for 3 days. The percentages of the CSC populations (n=3, mean±s.d.; Student’st-test) and the expression of RELB, an indicator of NF-κB activation, with or without TNFα for 24 h. (j) Cells were cultured with or without 10 ng ml−1TNFα for 3 days and analysed using the sphere-formation assay (n=3, mean±s.d.; Student’st-test). (k) The indicated numbers of cells were transplanted into the mammary fat pads of NOD/SCID mice. For 10 weeks, the mice were examined weekly for tumours by palpation. Statistically significant differences in tumorigenicity between the control and NF-κB-modified cells were determined using Fisher’s exact test. All data are representative of three independent experiments. NS, not significant. *P<0.05, **P<0.01 and ***P<0.001 (d–j). Figure 1: NF -κ B regulates the CSC population in basal-like breast cancer cell lines. ( a ) The correlation between constitutive NF-κB activation and the CD24 − /CD44 high /EpCAM + CSC population in various breast cancer cell lines. A linear regression analysis of values derived from the basal-like cell lines is shown as a dotted line ( n =3, mean±s.d., P =0.011; Pearson’s correlation coefficient). Relative NF-κB activities were determined as described in Methods. ( b ) The correlation between constitutive NF-κB activation and the ALDEFLUOR + CSC population in various breast cancer cell lines. A linear regression analysis of values derived from the basal-like cell lines is shown as a dotted line ( n =3, mean±s.d., P =0.015; Pearson’s correlation coefficient). ( c ) EMSA of NF-κB activation in control, IκBαSR and IKKβ-expressing breast cancer cells. ( d ) The percentages of the CD24 − /CD44 high /EpCAM + CSC populations ( n =3, mean±s.d. ; Student’s t -test) in basal-like cell lines with various NF-κB activation levels. ( e , f ) The percentages of the ALDEFLUOR + CSC populations ( n =3, mean±s.d. ; Student’s t -test) in the claudin-low ( e ) and luminal-like ( f ) cell lines with various levels of NF-κB activation. ( g , h ) NF-κB regulates the sphere-forming ability of basal-like cells ( g ), but not that of claudin-low and luminal-like cell lines ( h ); images showing sphere formation. Scale bar, 500 μm. ( i ) Fluorescence-activated cell sorting analysis of the CSC population in basal-like cell lines with or without TNFα treatment (10 ng ml −1 ) for 3 days. The percentages of the CSC populations ( n =3, mean±s.d. ; Student’s t -test) and the expression of RELB, an indicator of NF-κB activation, with or without TNFα for 24 h. ( j ) Cells were cultured with or without 10 ng ml −1 TNFα for 3 days and analysed using the sphere-formation assay ( n =3, mean±s.d. ; Student’s t -test). ( k ) The indicated numbers of cells were transplanted into the mammary fat pads of NOD/SCID mice. For 10 weeks, the mice were examined weekly for tumours by palpation. Statistically significant differences in tumorigenicity between the control and NF-κB-modified cells were determined using Fisher’s exact test. All data are representative of three independent experiments. NS, not significant. * P <0.05, ** P <0.01 and *** P <0.001 ( d – j ). Full size image NF-κB in non-CSCs is crucial in regulating CSC population To elucidate the molecular mechanisms of the NF-κB-mediated regulation of the CSC population, we first compared the NF-κB activities in the CSC and non-CSC fractions. Each cell fraction was isolated from two basal-like cells, MB468 and HCC1937 ( Fig. 2a ). Electrophoretic mobility shift assays (EMSAs) revealed that the NF-κB activities in the CSC and non-CSC fractions were indistinguishable in both cell lines ( Fig. 2b ), leading us to hypothesize that NF-κB activation in non-CSCs may regulate the CSC population. This hypothesis is in contrast to a previously proposed model, in which NF-κB activation in CSCs cell-autonomously maintains stemness [12] , [13] , [14] , [15] . To test this hypothesis, three basal-like cell lines with intact NF-κB activation were labelled with green fluorescent protein (GFP) and then co-cultured with a 10-fold excess of an unlabelled corresponding cell line that was engineered to confer modulated NF-κB activation ( Fig. 2c ). Following the co-culture, the populations of GFP + CSCs among all of the GFP + cells were measured. The co-culture containing the high-NF-κB cells displayed marked expansion of the GFP + CSC population, whereas a significant reduction in the GFP + CSC population was observed in the co-culture containing the low-NF-κB cells ( Fig. 2d ). Moreover, compared with GFP + cells sorted after co-culture with cells displaying intact NF-κB activation, the GFP + cells sorted after co-culture with high-NF-κB cells or low-NF-κB cells showed higher and lower mammosphere-formation activities, respectively ( Fig. 2e ). Based on the EMSAs of the GFP + and GFP − cells isolated after the co-culture, the NF-κB activation levels of the GFP + cells were not significantly affected by their co-culture, with the GFP − cells displaying different levels of NF-κB activation ( Fig. 2f ). This result indicates that the level of NF-κB activation in CSCs is not critical for the regulation of the CSC population. Furthermore, the result demonstrates that the non-labelled high- or low-NF-κB cells (the vast majority of which are non-CSCs) stimulate neighbouring CSCs in trans to regulate the CSC population without affecting CSC NF-κB activation levels. These findings reveal a non-cell-autonomous role for NF-κB in the regulation of the CSC population. The trans-stimulation by non-CSCs was significantly reduced when the GFP + cells were cultured separately from the high-NF-κB cells in trans-well chambers ( Fig. 2g ), indicating the requirement for direct cell–cell contact between the GFP + cells and the high-NF-κB cells to promote the efficient regulation of the CSC population. Nevertheless, because partial CSC population expansion was observed in the absence of cell–cell contact ( Fig. 2g ), we tested the involvement of IL-6 and IL-8, soluble cytokines that are known to be induced by NF-κB and regulate the CSC population [22] , [24] , in this partial effect. Neither IL-6 nor IL-8 induced the expansion of the CSC population and enhanced sphere formation in the basal-like cell lines ( Fig. 2h , Supplementary Fig. S4 ). Neutralizing antibodies against IL-6 and IL-8 could not inhibit the TNFα-induced or IKKβ-mediated expansion of the CSC population and enhancement of sphere formation ( Fig. 2i , Supplementary Fig. S4 ). These results indicate that the cell–cell contact-independent CSC expansion is not mediated by IL-6 or IL-8. 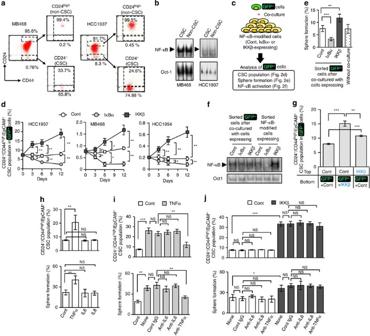Figure 2: Non-cell-autonomous role of NF-κB in the regulation of CSC populations of basal-like cell lines. (a) Characterization of CSC and non-CSC fractions. CSC and non-CSC fractions of MB468 and HCC1937 cells were isolated according to their CD24, CD44 and EpCAM expression levels. (b) Nuclear extracts were prepared from the sorted CSC and non-CSC populations presented inaand subjected to EMSAs. Arrows indicate the specific NF-κB/DNA complexes. (c–f) NF-κB regulates the CSC populationin trans. Schematic representation of the protocol for the co-culture assay (c). GFP-labelled cells were co-cultured with a 10-fold excess of cells with modified NF-κB activation. Following the indicated number of days of co-culture, the CSC populations of the GFP-labelled cells (n=3, mean±s.d.; Student’st-test) were measured (d). After 12 days of co-culture, the GFP-labelled cells were sorted and evaluated for sphere-forming ability (n=3, mean±s.d.; Student’st-test) (e); nuclear extracts were then prepared from the GFP-labelled and unlabelled cells for the EMSAs (f). (g) Contact between the GFP-labelled and IKKβ-expressing cells was required for the efficient expansion of the CSC population of GFP-labelled cells. GFP-labelled cells in the bottom chamber were co-cultured with control cells alone or with IKKβ-expressing cells in the same or the top chamber. After 3 days of co-culture, the CSC populations of GFP-labelled cells (n=3, mean±s.d.; Student’st-test) in the bottom chamber were determined. (h) HCC1937 cells were untreated or treated with IL-6 (50 ng ml−1), IL-8 (100 ng ml−1) or TNFα (10 ng ml−1) for 3 days and then subjected to fluorescence-activated cell sorting (FACS) analysis and sphere-formation assay (n=3, mean±s.d.; Student’st-test). (i) HCC1937 cells were treated with TNFα (10 ng ml−1) for 3 days in the presence of various neutralizing antibodies (2 μg ml−1) and then subjected to FACS analysis and sphere-formation assay (n=3, mean±s.d.; Student’st-test). (j) Control or IKKβ-expressing HCC1937 cells were treated with various neutralizing antibodies (2 μg ml−1) for 3 days and subjected to FACS analysis and sphere-formation assay (n=3, mean±s.d.; Student’st-test). All data are representative of three independent experiments. NS, not significant. *P<0.05, **P<0.01 and ***P<0.001 (d,e,g–j). Figure 2: Non-cell-autonomous role of NF -κ B in the regulation of CSC populations of basal-like cell lines. ( a ) Characterization of CSC and non-CSC fractions. CSC and non-CSC fractions of MB468 and HCC1937 cells were isolated according to their CD24, CD44 and EpCAM expression levels. ( b ) Nuclear extracts were prepared from the sorted CSC and non-CSC populations presented in a and subjected to EMSAs. Arrows indicate the specific NF-κB/DNA complexes. ( c – f ) NF-κB regulates the CSC population in trans . Schematic representation of the protocol for the co-culture assay ( c ). GFP-labelled cells were co-cultured with a 10-fold excess of cells with modified NF-κB activation. Following the indicated number of days of co-culture, the CSC populations of the GFP-labelled cells ( n =3, mean±s.d. ; Student’s t -test) were measured ( d ). After 12 days of co-culture, the GFP-labelled cells were sorted and evaluated for sphere-forming ability ( n =3, mean±s.d. ; Student’s t -test) ( e ); nuclear extracts were then prepared from the GFP-labelled and unlabelled cells for the EMSAs ( f ). ( g ) Contact between the GFP-labelled and IKKβ-expressing cells was required for the efficient expansion of the CSC population of GFP-labelled cells. GFP-labelled cells in the bottom chamber were co-cultured with control cells alone or with IKKβ-expressing cells in the same or the top chamber. After 3 days of co-culture, the CSC populations of GFP-labelled cells ( n =3, mean±s.d. ; Student’s t -test) in the bottom chamber were determined. ( h ) HCC1937 cells were untreated or treated with IL-6 (50 ng ml −1 ), IL-8 (100 ng ml −1 ) or TNFα (10 ng ml −1 ) for 3 days and then subjected to fluorescence-activated cell sorting (FACS) analysis and sphere-formation assay ( n =3, mean±s.d. ; Student’s t -test). ( i ) HCC1937 cells were treated with TNFα (10 ng ml −1 ) for 3 days in the presence of various neutralizing antibodies (2 μg ml −1 ) and then subjected to FACS analysis and sphere-formation assay ( n =3, mean±s.d. ; Student’s t -test). ( j ) Control or IKKβ-expressing HCC1937 cells were treated with various neutralizing antibodies (2 μg ml −1 ) for 3 days and subjected to FACS analysis and sphere-formation assay ( n =3, mean±s.d. ; Student’s t -test). All data are representative of three independent experiments. NS, not significant. * P <0.05, ** P <0.01 and *** P <0.001 ( d , e , g – j ). Full size image JAG1 is an NF-κB-inducible NOTCH ligand To identify molecules that mediate the cell–cell interactions involved in NF-κB-dependent CSC regulation, we focused on the NOTCH signal because NOTCH reportedly transduces signals that maintain the CSC population in breast cancer [25] , [26] , [27] . Expression of the NOTCH target genes HEY1 and HEY2 in CSCs was higher than that in non-CSCs ( Fig. 3a ). Moreover, HEY1 and HEY2 expression in CSCs was markedly enhanced by elevated NF-κB activation, but was not significantly affected in non-CSCs ( Fig. 3a ). These results suggest that the NOTCH signalling in CSCs is more highly activated than that in non-CSCs and that NF-κB activation further enhances NOTCH activation in CSCs. Given the lack of increase in NOTCH family expression following enhanced NF-κB activation in either the CSC or non-CSC population ( Supplementary Fig. S5 ), these results led us to hypothesize that the non-cell-autonomous function of NF-κB is mediated by NOTCH ligands expressed in non-CSCs. The high-NF-κB cells showed enhanced JAG1 mRNA and protein expression; however, the expression levels were significantly reduced in the low-NF-κB cells ( Fig. 3b ). TNFα stimulation also induced JAG1 mRNA and protein expression ( Fig. 3d ). Interestingly, the expression levels of other NOTCH ligands were not significantly affected by NF-κB activation ( Fig. 3b ). Furthermore, TNFα stimulation did not induce the mRNA or protein expression of JAG1 in either the luminal-like or claudin-low cells, although the induction of RELB , a known NF-κB-inducible gene, was clearly observed ( Fig. 3f ). These results indicate that JAG1 is the only NF-κB-regulated NOTCH ligand gene in the basal-like cell lines. Further, this NF-κB-dependent JAG1 expression is likely specific to the basal-like subtype. 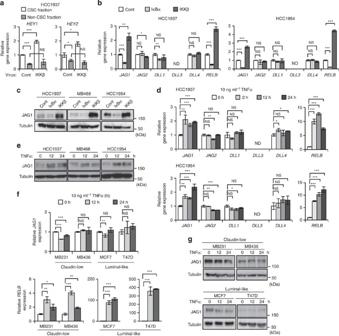Figure 3: JAG1 is a unique NF-κB-inducible NOTCH ligand in basal-like breast cancers. (a)HEY1andHEY2mRNA expression levels in CSCs are higher than in the non-CSC population and are further enhanced by NF-κB activation in HCC1937 cells. Total RNA fractions were prepared from CSC and non-CSC cells, and a real-time reverse transcriptase PCR (RT–PCR) analysis was performed (n=3, mean±s.d.; Student’st-test). (b) Real-time RT–PCR analysis of NOTCH ligands andRELBmRNA expression (n=3, mean±s.d.; Student’st-test) in control, IκBαSR and IKKβ-expressing cells was performed in two basal-like cell lines. (c) Western blotting analyses of JAG1 protein regulated by NF-κB. (d) Real-time PCR analysis of NOTCH ligands and ofRELBmRNA expression (n=3, mean±s.d.; Student’st-test) in TNFα-treated basal-like subtype cells. (e) Western blotting analyses of JAG1 protein induced by TNFα treatment. (f) Real-time PCR analysis ofJAG1andRELBmRNA expression (n=3, mean±s.d.; Student’st-test) in cells treated with 10 ng ml−1TNFα for the indicated times. (g) Western blotting of JAG1 expression in cells treated with 10 ng ml−1TNFα for the indicated times. All data are representative of three independent experiments. ND, not detected; NS, not significant. *P<0.05, **P<0.01 and ***P<0.001 (a,b,d,f). Figure 3: JAG1 is a unique NF -κ B-inducible NOTCH ligand in basal-like breast cancers. ( a ) HEY1 and HEY2 mRNA expression levels in CSCs are higher than in the non-CSC population and are further enhanced by NF-κB activation in HCC1937 cells. Total RNA fractions were prepared from CSC and non-CSC cells, and a real-time reverse transcriptase PCR (RT–PCR) analysis was performed ( n =3, mean±s.d. ; Student’s t -test). ( b ) Real-time RT–PCR analysis of NOTCH ligands and RELB mRNA expression ( n =3, mean±s.d. ; Student’s t -test) in control, IκBαSR and IKKβ-expressing cells was performed in two basal-like cell lines. ( c ) Western blotting analyses of JAG1 protein regulated by NF-κB. ( d ) Real-time PCR analysis of NOTCH ligands and of RELB mRNA expression ( n =3, mean±s.d. ; Student’s t -test) in TNFα-treated basal-like subtype cells. ( e ) Western blotting analyses of JAG1 protein induced by TNFα treatment. ( f ) Real-time PCR analysis of JAG1 and RELB mRNA expression ( n =3, mean±s.d. ; Student’s t -test) in cells treated with 10 ng ml −1 TNFα for the indicated times. ( g ) Western blotting of JAG1 expression in cells treated with 10 ng ml −1 TNFα for the indicated times. All data are representative of three independent experiments. ND, not detected; NS, not significant. * P <0.05, ** P <0.01 and *** P <0.001 ( a , b , d , f ). Full size image JAG1 mediates NF-κB-mediated stimulation of CSCs by non-CSCs To address whether JAG1 mediates trans signalling, we first generated basal-like cells overexpressing JAG1 ( Fig. 4a ). JAG1 overexpression resulted in an expansion of the CSC population ( Fig. 4b ). The co-culture of GFP + cells with JAG1-overexpressing cells resulted in both CSC population expansion ( Fig. 4c ) and enhanced mammosphere formation ( Fig. 4d ) in the GFP + cells. Furthermore, enhanced JAG1 expression elevated HEY1 and HEY2 expression ( Fig. 4e ). To further analyse the critical role of JAG1, we reduced endogenous JAG1 expression. CSC population expansion was significantly reduced in the high-NF-κB cells in response to JAG1 silencing, whereas JAG1 silencing did not affect NF-κB activation, as evidenced by the efficient RELB induction ( Fig. 4f ). The TNFα-induced CSC population expansion was also significantly reduced by JAG1 silencing ( Fig. 4h ). Moreover, the complementation of the JAG1-silenced cells with JAG1 abolished the shJAG1-mediated inhibition of TNFα stimulation-induced CSC expansion ( Fig. 4j ). These results clearly indicate that NF-κB-induced JAG1 expression in non-CSCs has a critical role in CSC expansion. To further confirm the requirement for NOTCH signalling in NF-κB-mediated trans signalling, we analysed the effect of γ-secretase inhibitors (GSIs) and the knockdown of RBPJ, a component of the transcription complex that is essential for NOTCH target gene expression [28] , [29] , [30] , on NF-κB-induced CSC expansion. Both the GSIs and RBPJ-silencing significantly blocked the TNFα- and NF-κB-induced CSC population expansion ( Fig. 4l–q , Supplementary Fig. S6 ). 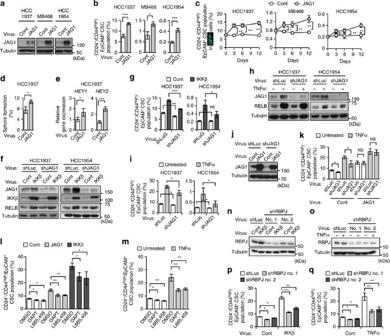Figure 4: JAG1 is crucial in the NF-κB-mediated stimulation of CSCs by non-CSCs. (a) Western blotting analyses of JAG1 expression in JAG1-overexpressing cells. (b) Flow-cytometry analysis of the CSC populations (n=3, mean±s.d.; Student’st-test) in JAG1-overexpressing cells. (c,d) GFP-labelled cells were co-cultured with a 10-fold excess of control or JAG1-overexpressing cells. After the co-culture, the CSC populations (n=3, mean±s.d.; Student’st-test) of the GFP-labelled cells were measured by flow-cytometry analysis (c). After 12 days of co-culture, the GFP-labelled cells were sorted and analysed for sphere-forming ability (n=3, mean±s.d.; Student’st-test) (d). (e)HEY1andHEY2mRNA expression (n=3, mean±s.d.; Student’st-test) in JAG1-overexpressing cells. (f) Western blotting of whole-cell lysates derived from control or IKKβ-overexpressing basal-like cells that additionally express either shLuc or shJAG1 (shLuc; control short hairpin RNA against luciferase gene). (g) Flow-cytometry analysis of the basal-like cells depicted inf(n=3, mean±s.d.; Student’st-test). (h) Western blotting analysis of whole-cell lysates derived from TNFα-treated basal-like cells that express either shLuc or shJAG1. (i) Basal-like cells expressing either shLuc or shJAG1 were untreated or treated with TNFα10 ng ml−1for 3 days, and then CSC populations (n=3, mean±s.d.; Student’st-test) were measured by flow-cytometry analysis. (j) Western blotting analyses of JAG1 expression in shLuc- or shJAG1-expressing HCC1937 cells that were further complemented with JAG1. (k) The HCC1937 cells analysed injwere untreated or treated with TNFα (10 ng ml−1) for 3 days, and then CSC populations (n=3, mean±s.d.; Student’st-test) were measured by flow-cytometry analysis. (l,m) Control, JAG1-expressing, IKKβ-expressing (l) and TNFα-treated (m) HCC1937 cells were untreated or treated withN-[N-(3,5-difluorophenacetyl)-L-alanyl]-S-phenylglycine t-butyl ester (DAPT) (5 μM) or L685,458 (10 μM) for 3 days, and then CSC populations (n=3, mean±s.d.; Student’st-test) were measured by flow-cytometry analysis. (n,o) Western blotting of whole-cell lysates derived from IKKβ-overexpressing (n) and TNFα-treated (o) HCC1937 cells that further express shLuc or shRBPJ. (p,q) Flow-cytometry analysis of the HCC1937 cells depicted innando(n=3, mean±s.d.; Student’st-test). All data are representative of three independent experiments. NS, not significant. *P<0.05, **P<0.01 and ***P<0.001 (b–e,g,i,k–m,p,q). Figure 4: JAG1 is crucial in the NF -κ B-mediated stimulation of CSCs by non-CSCs. ( a ) Western blotting analyses of JAG1 expression in JAG1-overexpressing cells. ( b ) Flow-cytometry analysis of the CSC populations ( n =3, mean±s.d. ; Student’s t -test) in JAG1-overexpressing cells. ( c , d ) GFP-labelled cells were co-cultured with a 10-fold excess of control or JAG1-overexpressing cells. After the co-culture, the CSC populations ( n =3, mean±s.d. ; Student’s t -test) of the GFP-labelled cells were measured by flow-cytometry analysis ( c ). After 12 days of co-culture, the GFP-labelled cells were sorted and analysed for sphere-forming ability ( n =3, mean±s.d. ; Student’s t -test) ( d ). ( e ) HEY1 and HEY2 mRNA expression ( n =3, mean±s.d. ; Student’s t -test) in JAG1-overexpressing cells. ( f ) Western blotting of whole-cell lysates derived from control or IKKβ-overexpressing basal-like cells that additionally express either shLuc or shJAG1 (shLuc; control short hairpin RNA against luciferase gene). ( g ) Flow-cytometry analysis of the basal-like cells depicted in f ( n =3, mean±s.d. ; Student’s t -test). ( h ) Western blotting analysis of whole-cell lysates derived from TNFα-treated basal-like cells that express either shLuc or shJAG1. ( i ) Basal-like cells expressing either shLuc or shJAG1 were untreated or treated with TNFα10 ng ml −1 for 3 days, and then CSC populations ( n =3, mean±s.d. ; Student’s t -test) were measured by flow-cytometry analysis. ( j ) Western blotting analyses of JAG1 expression in shLuc- or shJAG1-expressing HCC1937 cells that were further complemented with JAG1. ( k ) The HCC1937 cells analysed in j were untreated or treated with TNFα (10 ng ml −1 ) for 3 days, and then CSC populations ( n =3, mean±s.d. ; Student’s t -test) were measured by flow-cytometry analysis. ( l , m ) Control, JAG1-expressing, IKKβ-expressing ( l ) and TNFα-treated ( m ) HCC1937 cells were untreated or treated with N -[ N -(3,5-difluorophenacetyl)- L -alanyl] -S- phenylglycine t-butyl ester (DAPT) (5 μM) or L685,458 (10 μM) for 3 days, and then CSC populations ( n =3, mean±s.d. ; Student’s t -test) were measured by flow-cytometry analysis. ( n , o ) Western blotting of whole-cell lysates derived from IKKβ-overexpressing ( n ) and TNFα-treated ( o ) HCC1937 cells that further express shLuc or shRBPJ. ( p , q ) Flow-cytometry analysis of the HCC1937 cells depicted in n and o ( n =3, mean±s.d. ; Student’s t -test). All data are representative of three independent experiments. NS, not significant. * P <0.05, ** P <0.01 and *** P <0.001 ( b – e , g , i , k – m , p , q ). Full size image NF-κB-JAG1 axis is unique to the basal-like subtype in vivo To determine whether the aforementioned functional link between NF-κB and NOTCH signalling in breast cancer cell lines can be applied to human breast cancer in vivo , 534 breast tumours from The Cancer Genome Atlas [31] were categorized into basal-like, claudin-low, ERBB2-enriched and luminal-like subtypes based on a hierarchical clustering analysis of their gene expression profiles ( Supplementary Fig. S7 ). We then tested whether the NF-κB-target genes were highly expressed in the basal-like and claudin-low subtypes. Twenty-eight genes were chosen as NF-κB-dependent genes because their expression levels were induced by TNFα stimulation and repressed by IκBαSR expression in human HeLa cell lines [32] . A Gene Set Enrichment Analysis (GSEA) [33] , [34] revealed that the NF-κB-dependent genes were highly expressed in the basal-like subtype when compared with the ERBB2-enriched and luminal-like subtypes, but this difference was not significant when compared with the claudin-low subtype ( Fig. 5a ). Similarly, the NF-κB-dependent genes were highly expressed in the claudin-low subtype when compared with the ERBB2-enriched and luminal-like subtypes ( Fig. 5b ). These data strongly suggest that NF-κB is highly activated in basal-like and claudin-low subtype tumours, which is consistent with our findings in the cell lines ( Fig. 1a ). We next investigated the relationship between NF-κB activation and JAG1 expression. GSEA was performed with the NF-κB-dependent gene set and the set of genes whose expression levels were correlated with JAG1 expression in each subtype. The expression of the NF-κB-dependent gene set was significantly correlated with JAG1 expression ( Fig. 5c ), but not with the expression of other NOTCH ligands ( Fig. 5d ), in the basal-like subtype. These results strongly suggest that JAG1 is a unique gene that is specifically regulated by NF-κB in basal-like breast tumours. Because CSCs are primarily responsible for the formation of tumour metastases, we next analysed the relationship between the expression levels of various NOTCH ligands and the metastasis-free survival rates using the same database ( Supplementary Fig. S7 ). JAG1 expression was significantly correlated with a short metastasis-free survival only in the basal-like breast tumour subtype ( Fig. 5e ). An Extraction of Expression Module analysis [35] of the same clinical data also revealed that the strong NF-κB activation and the NF-κB-JAG1 axis were specific to the basal-like subtype ( Supplementary Fig. S8 ). The analyses of these clinical data strongly support our hypothesis that JAG1 has a basal-like subtype-specific role in the maintenance of the CSC population. 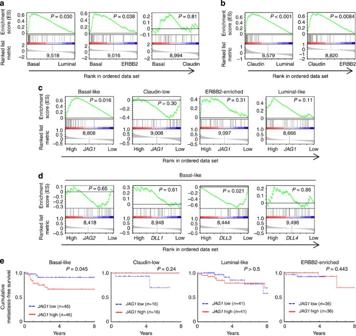Figure 5: Correlation between NF-κB-JAG1 signalling and patient survival. (a) Strong NF-κB activation in basal-like subtype of breast cancer. A GSEA was performed to determine whether the NF-κB-dependent gene set reported previously32(Supplementary Table S2) was highly expressed in the basal-like subtype of breast cancer compared with other subtypes. All of the genes (n=17,814) on the microarray were ranked according to their differential expression levels across the two subtypes using a signal-to-noise metric. TheP-values were determined by a random permutation test. (b) Strong NF-κB activation in the claudin-low subtype of breast cancer. GESA was performed as ina, except that expression of the NF-κB-dependent gene set in the claudin-low subtype of breast cancer was compared with that in the luminal-like and ERBB2-enriched subtypes of breast cancer. (c)JAG1expression is significantly correlated with NF-κB activation in a basal-like subtype-specific manner. GSEA was performed to determine whether the NF-κB-dependent gene set was correlated withJAG1expression in various breast cancer subtypes. All of the genes on the microarray were ranked according to their correlation withJAG1expression using the Pearson’s correlation metric. TheP-values were determined by a random permutation test. (d) Lack of positive correlation between NF-κB activation and the expression of other NOTCH ligands in the basal-like subtype of breast cancer. GSEA was used to determine whether the NF-κB-dependent gene set was correlated with the expression of each NOTCH ligand in the basal-like subtype of breast cancer. All of the genes on the microarray were ranked according to their correlation with the expression of each NOTCH ligand using the Pearson’s correlation metric. TheP-values were determined by a random permutation test. (e) Kaplan–Meier curves showing the relation between cumulative metastasis-free survival and the expression levels ofJAG1in patients with various subtypes of breast cancer. Statistical differences between pairs of metastasis-free survival curves were calculated using a log-rank test. Numbers shown in the ‘ranked list metric’ column ofa–dindicate the ranking of the gene whose ranking metric score is zero. Figure 5: Correlation between NF -κ B-JAG1 signalling and patient survival. ( a ) Strong NF-κB activation in basal-like subtype of breast cancer. A GSEA was performed to determine whether the NF-κB-dependent gene set reported previously [32] ( Supplementary Table S2 ) was highly expressed in the basal-like subtype of breast cancer compared with other subtypes. All of the genes ( n =17,814) on the microarray were ranked according to their differential expression levels across the two subtypes using a signal-to-noise metric. The P -values were determined by a random permutation test. ( b ) Strong NF-κB activation in the claudin-low subtype of breast cancer. GESA was performed as in a , except that expression of the NF-κB-dependent gene set in the claudin-low subtype of breast cancer was compared with that in the luminal-like and ERBB2-enriched subtypes of breast cancer. ( c ) JAG1 expression is significantly correlated with NF-κB activation in a basal-like subtype-specific manner. GSEA was performed to determine whether the NF-κB-dependent gene set was correlated with JAG1 expression in various breast cancer subtypes. All of the genes on the microarray were ranked according to their correlation with JAG1 expression using the Pearson’s correlation metric. The P -values were determined by a random permutation test. ( d ) Lack of positive correlation between NF-κB activation and the expression of other NOTCH ligands in the basal-like subtype of breast cancer. GSEA was used to determine whether the NF-κB-dependent gene set was correlated with the expression of each NOTCH ligand in the basal-like subtype of breast cancer. All of the genes on the microarray were ranked according to their correlation with the expression of each NOTCH ligand using the Pearson’s correlation metric. The P -values were determined by a random permutation test. ( e ) Kaplan–Meier curves showing the relation between cumulative metastasis-free survival and the expression levels of JAG1 in patients with various subtypes of breast cancer. Statistical differences between pairs of metastasis-free survival curves were calculated using a log-rank test. Numbers shown in the ‘ranked list metric’ column of a – d indicate the ranking of the gene whose ranking metric score is zero. Full size image NIK induces JAG1 expression in some breast cancer cell lines Because TNFα stimulation induced JAG1 expression, JAG1 is induced by the canonical NF-κB pathway. However, the expression of IκBαSR or IKKβ altered the level of nuclear RELB, an NF-κB subunit activated by the non-canonical pathway, in addition to nuclear RELA ( Fig. 6a ). Moreover, we previously reported that basal-like cell lines show higher NIK mRNA expression levels than luminal-like cell lines and that enhanced NIK mRNA expression results in the accumulation and activation of NIK protein, leading to the constitutive activation of NF-κB [5] , [36] . Given that NIK is an activator of IKKα in the non-canonical pathway, these results led us to hypothesize that enhanced NIK expression-induced non-canonical pathway activation may affect JAG1 expression. Because NIK protein is barely detectable due to its proteasome-mediated degradation [37] , we used proteasome inhibitor MG132 to stabilize NIK so that we could analyse the effect of NIK silencing. NIK silencing resulted in the significant reduction of JAG1 expression in two basal-like cell lines, HCC1937 and HCC1143 ( Fig. 6b ). Furthermore, NIK silencing resulted in the significant reduction of the CSC population ( Fig. 6d ). Because NIK silencing resulted in the significant reduction of nuclear RELB, but not RELA, in these two basal-like cell lines ( Fig. 6e ), JAG1 expression is likely regulated by the non-canonical pathway in addition to the canonical pathway. Therefore, the level of total NF-κB activation (the sum of canonical and non-canonical activation) may determine the level of JAG1 expression in basal-like cells. Consistent with this hypothesis, NIK silencing resulted in the significant reduction of total NF-κB activation in the HCC1937 and HCC1143 cell lines ( Fig. 6c ), whereas NIK silencing minimally affected the levels of nuclear RELA and RELB, total NF-κB activation, JAG1 expression and the CSC population in the HCC38 cell line ( Fig. 6e–h ), even though all three of these cell lines highly express the NIK gene [5] . Thus, the contribution of NIK to total NF-κB activation and JAG1 induction varies among basal-like cell lines and, perhaps, among the clinical samples of the basal-like breast cancers. 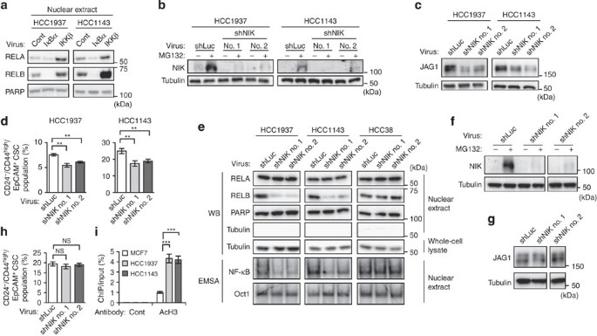Figure 6: NIK mediates JAG1 expression in a subset of basal-like breast cancer cells. (a) Western blotting analyses of RELA and RELB levels in nuclear extracts of control, IκBαSR- and IKKβ-expressing HCC1937 and HCC1143 cells. (b) NIK expression in HCC1937 and HCC1143 cells expressing shLuc, shNIK no. 1 or shNIK no. 2. HCC1937 and HCC1143 cells expressing shLuc, shNIK no. 1 or shNIK no. 2 were either untreated or treated with MG132 (10 μM) for 2 h. Whole-cell lysates prepared with or without MG132 treatment were subjected to western blotting. (c) Western blotting analyses of JAG1 expression in HCC1937 and HCC1143 cells expressing shLuc, shNIK no. 1 or shNIK no. 2. (d) The CSC populations (n=3, mean±s.d.; Student’st-test) were determined by flow-cytometry analysis. (e) RELA and RELB expression and NF-κB activation in nuclear extracts of shLuc-, shNIK no. 1- or shNIK no. 2-expressing cells. Nuclear extracts were subjected to western blotting and EMSA. Whole-cell lysates were analysed as a positive control for detection of tubulin. (f) NIK expression in HCC38 cells expressing shLuc, shNIK no. 1 or shNIK no. 2. Cells expressing shLuc, shNIK no. 1 or shNIK no. 2 were either untreated or treated with MG132 (10 μM) for 2 h. Whole-cell lysates prepared with or without MG132 treatment were subjected to western blotting. (g) Western blotting analyses of JAG1 expression in HCC38 cells expressing shLuc, shNIK no. 1 or shNIK no. 2. (h) The CSC populations (n=3, mean±s.d.; Student’st-test) were determined by flow-cytometry analysis. (i) The histone H3 acetylation profile in theNIKpromoter region (n=3, mean±s.d.; Student’st-test) was analysed using a chromatin immunoprecipitation (ChIP) assay in luminal-like (MCF7) and basal-like (HCC1937 and HCC1143) cell lines. All data are representative of three independent experiments. NS, not significant. **P<0.01 and ***P<0.001 (d,h,i). Figure 6: NIK mediates JAG1 expression in a subset of basal-like breast cancer cells. ( a ) Western blotting analyses of RELA and RELB levels in nuclear extracts of control, IκBαSR- and IKKβ-expressing HCC1937 and HCC1143 cells. ( b ) NIK expression in HCC1937 and HCC1143 cells expressing shLuc, shNIK no. 1 or shNIK no. 2. HCC1937 and HCC1143 cells expressing shLuc, shNIK no. 1 or shNIK no. 2 were either untreated or treated with MG132 (10 μM) for 2 h. Whole-cell lysates prepared with or without MG132 treatment were subjected to western blotting. ( c ) Western blotting analyses of JAG1 expression in HCC1937 and HCC1143 cells expressing shLuc, shNIK no. 1 or shNIK no. 2. ( d ) The CSC populations ( n =3, mean±s.d. ; Student’s t -test) were determined by flow-cytometry analysis. ( e ) RELA and RELB expression and NF-κB activation in nuclear extracts of shLuc-, shNIK no. 1- or shNIK no. 2-expressing cells. Nuclear extracts were subjected to western blotting and EMSA. Whole-cell lysates were analysed as a positive control for detection of tubulin. ( f ) NIK expression in HCC38 cells expressing shLuc, shNIK no. 1 or shNIK no. 2. Cells expressing shLuc, shNIK no. 1 or shNIK no. 2 were either untreated or treated with MG132 (10 μM) for 2 h. Whole-cell lysates prepared with or without MG132 treatment were subjected to western blotting. ( g ) Western blotting analyses of JAG1 expression in HCC38 cells expressing shLuc, shNIK no. 1 or shNIK no. 2. ( h ) The CSC populations ( n =3, mean±s.d. ; Student’s t -test) were determined by flow-cytometry analysis. ( i ) The histone H3 acetylation profile in the NIK promoter region ( n =3, mean±s.d. ; Student’s t -test) was analysed using a chromatin immunoprecipitation (ChIP) assay in luminal-like (MCF7) and basal-like (HCC1937 and HCC1143) cell lines. All data are representative of three independent experiments. NS, not significant. ** P <0.01 and *** P <0.001 ( d , h , i ). Full size image We have previously reported that the treatment of luminal-like cells with a histone deacetylase inhibitor increased NIK mRNA expression, whereas the same treatment of basal-like cells did not show this effect [36] . Furthermore, histone H3 acetylation in the 5′ regulatory region of the NIK promoter was significantly higher in the two basal-like cell lines compared with luminal-like MCF7 cells ( Fig. 6i ). These results strongly suggest that in some of the basal-like cell lines, epigenetically induced NIK expression has a critical role in NF-κB-induced JAG1 expression in non-CSCs, which could lead to CSC population expansion. Therefore, the NIK-NF-κB-JAG1-NOTCH axis may establish an intratumoural niche that regulates the CSC population in a subset of basal-like breast tumours in vivo . NOTCH expands CSC population only in the basal-like subtype We next addressed whether normal cells that constitute tumour microenvironments express JAG1 in an NF-κB-dependent manner. First, the expression of JAG1 (but not other NOTCH ligands) was induced in macrophages either by lipopolysaccharide treatment or by the ectopic expression of IKKβEE ( Fig. 7a–d ). Second, the expression of JAG1 (but not other NOTCH ligands) was induced in mammary fibroblasts either by TNFα treatment or by the ectopic expression of IKKβEE ( Fig. 7e–h ). In normal mammary gland development, PR induces RANK ligand expression in luminal epithelial cells [38] , [39] . RANK ligand then stimulates RANK in mammary stem cells (MaSCs) and basal myoepithelial cells to induce NF-κB activation, which promotes rapid cell growth that ultimately leads to mammary gland development. Interestingly, the treatment of mice with medroxyprogesterone acetate (MPA, a synthetic PR derivative) significantly induced JAG1 expression in basal myoepithelial cells ( Fig. 7i ). This result strongly suggests that RANK-induced NF-κB activation results in the induction of JAG1 expression in basal myoepithelial cells. 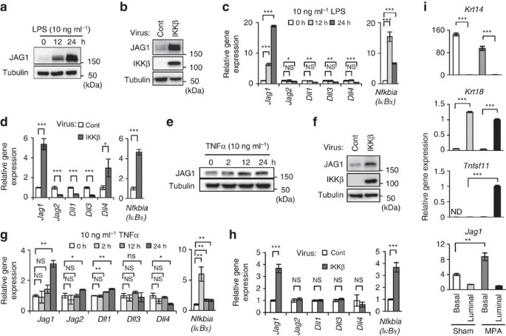Figure 7: NF-κB-dependent induction of JAG1 in cells of the tumour microenvironment. (a–d) Western blotting of JAG1 in bone marrow-derived macrophages stimulated with 10 ng ml−1lipopolysaccharide (LPS) (a) or with IKKβEE expression (b). Real-time reverse transcriptase PCR (RT–PCR) analysis of Notch ligands and IκBα (Nfkbia) mRNA expression (n=3, mean±s.d.; Student’st-test) in bone marrow-derived macrophages with LPS (c) or with IKKβEE expression (d). (e–h) Western blotting of JAG1 in immortalized mouse mammary fibroblast cells stimulated with 10 ng ml−1TNFα (e) or with IKKβEE expression (f). Real-time RT–PCR analysis of Notch ligands and IκBα (Nfkbia) mRNA expression (n=3, mean±s.d.; Student’st-test) in immortalized mouse mammary fibroblast cells with 10 ng ml−1TNFα (g) or with IKKβEE expression (h). (i) Mammary basal and luminal epithelial cells were isolated from 10-week-old female mice with or withoutin vivoMPA treatment for 3 weeks. A real-time RT–PCR analysis was performed to quantifyJag1,Krt14,Krt8andTnfsf11mRNA expression (n=3, mean±s.d.; Student’st-test). The induction ofNfkbiashown inc,d,gandhindicates NF-κB activation. All data are representative of three independent experiments. ND, not detected; NS, not significant. *P<0.05, **P<0.01 and ***P<0.001 (c,d,g–i). Figure 7: NF-κB-dependent induction of JAG1 in cells of the tumour microenvironment. ( a – d ) Western blotting of JAG1 in bone marrow-derived macrophages stimulated with 10 ng ml −1 lipopolysaccharide (LPS) ( a ) or with IKKβEE expression ( b ). Real-time reverse transcriptase PCR (RT–PCR) analysis of Notch ligands and IκBα ( Nfkbia ) mRNA expression ( n =3, mean±s.d. ; Student’s t -test) in bone marrow-derived macrophages with LPS ( c ) or with IKKβEE expression ( d ). ( e – h ) Western blotting of JAG1 in immortalized mouse mammary fibroblast cells stimulated with 10 ng ml −1 TNFα ( e ) or with IKKβEE expression ( f ). Real-time RT–PCR analysis of Notch ligands and IκBα ( Nfkbia ) mRNA expression ( n =3, mean±s.d. ; Student’s t -test) in immortalized mouse mammary fibroblast cells with 10 ng ml −1 TNFα ( g ) or with IKKβEE expression ( h ). ( i ) Mammary basal and luminal epithelial cells were isolated from 10-week-old female mice with or without in vivo MPA treatment for 3 weeks. A real-time RT–PCR analysis was performed to quantify Jag1 , Krt14 , Krt8 and Tnfsf11 mRNA expression ( n =3, mean±s.d. ; Student’s t -test). The induction of Nfkbia shown in c , d , g and h indicates NF-κB activation. All data are representative of three independent experiments. ND, not detected; NS, not significant. * P <0.05, ** P <0.01 and *** P <0.001 ( c , d , g – i ). Full size image To understand the effect of JAG1 expression on normal cells that constitute tumour microenvironments on CSC population regulation in breast cancer, we generated claudin-low and luminal-like cell lines that overexpressed JAG1. As observed in the JAG1-overexpressing basal-like cells, JAG1 overexpression resulted in the activation of NOTCH signalling as judged by the induction of NOTCH1 ICD ( Figs 4e and 8a ). However, NOTCH activation scarcely resulted in the expansion of the CSC population of the claudin-low and luminal-like cell lines when compared with that of the basal-like cell lines ( Figs 4b and 8b ). These results strongly suggest that the NOTCH-dependent CSC population expansion is specific to the basal-like subtype and that the tumour microenvironment generated by JAG1-expressing normal cells is likely to maintain the CSC population of basal-like breast cancer. 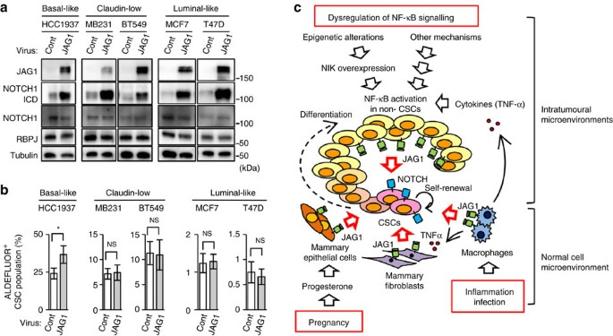Figure 8: JAG1-induced NOTCH activation expands the CSC population in a basal-like subtype-specific manner. (a) Western blotting of whole-cell lysates derived from control or JAG1-overexpressing basal-like, claudin-low and luminal-like cells was performed. (b) The percentages of the ALDEFLUOR+CSC population (n=3, mean±s.d.; Student’st-test) in control or JAG1-overexpressing cells were analysed. NS, not significant. *P<0.05. (c) A model illustrating the NF-κB-mediated maintenance of the CSC population of basal-like breast cancerin vivo. See text for details. All data are representative of three independent experiments. Figure 8: JAG1-induced NOTCH activation expands the CSC population in a basal-like subtype-specific manner. ( a ) Western blotting of whole-cell lysates derived from control or JAG1-overexpressing basal-like, claudin-low and luminal-like cells was performed. ( b ) The percentages of the ALDEFLUOR + CSC population ( n =3, mean±s.d. ; Student’s t -test) in control or JAG1-overexpressing cells were analysed. NS, not significant. * P <0.05. ( c ) A model illustrating the NF-κB-mediated maintenance of the CSC population of basal-like breast cancer in vivo . See text for details. All data are representative of three independent experiments. Full size image The involvement of NF-κB in the maintenance of the CSC population in breast cancer has been reported elsewhere [12] , [13] , [14] , [15] . Inhibition of NF-κB or IKKα activation results in the reduction of the CSC population of luminal-like breast cancer-generated MMTV-ErbB2 transgenic mice. However, the precise mechanisms by which NF-κB regulates CSC population remain unclear. On the other hand, the cell-autonomous role of NOTCH signalling in the maintenance of breast CSCs has been demonstrated [25] , [26] , [27] . Moreover, it has been reported that JAG1 is highly expressed in basal-like subtype [40] and that JAG1 expression correlates with poor outcome in breast cancer [41] , [42] . Therefore, it is critical to elucidate the functional interactions that occur between NF-κB and NOTCH signalling to regulate the CSC population. This study addresses this issue and demonstrates the non-cell-autonomous role of NF-κB in the activation of NOTCH signalling in CSCs. We propose a model by which NF-κB regulates the CSC population in basal-like breast cancers ( Fig. 8c ). The constitutive activation of NF-κB in basal-like breast cancer is significantly higher than that in the luminal-like subtype. This result could be attributed to enhanced NIK expression via subtype-specific epigenetic alterations [5] , [36] , some other dysregulation of NF-κB signalling caused by unknown mechanisms or inflammatory cytokines secreted from inflammatory infiltrates, such as macrophages. The cell-autonomous elevation of NF-κB activation induces JAG1 expression in a basal-like subtype-specific manner. Although JAG1 induction occurs in both CSC and non-CSC populations, the vast majority occurs in non-CSC populations. Therefore, intratumoural niches, which are primarily composed of JAG1-presenting non-CSCs, are formed and stimulate NOTCH signalling in CSCs to promote CSC self-renewal (the intratumoural microenvironments in Fig. 8c ). In addition, normal cells that constitute tumour microenvironments also express JAG1 in an NF-κB-dependent manner. The stimulation of Toll-like receptors, which is triggered by infection or inflammation, induces JAG1 and inflammatory cytokines, such as TNFα in macrophages. TNFα in turn stimulates JAG1 expression in mammary fibroblasts and cancer cells. Moreover, given that the MPA treatment of mice resulted in JAG1 induction in basal myoepithelial cells, the continuous production of PR during pregnancy may induce JAG1 expression in basal myoepithelial cells in humans, thus partly accounting for the increased incidence of pregnancy-associated breast cancer [43] . Therefore, in addition to non-CSC populations, JAG-expressing macrophages, fibroblasts and basal myoepithelial cells may form niches that regulate the self-renewal of CSCs in an NF-κB-dependent manner (the normal cell microenvironments in Fig. 8c ). Moreover, the NOTCH-dependent expansion of the CSC population may be specific to the basal-like subtype. Although the mechanism by which this specificity occurs remains unknown, some of the NOTCH target genes critical for CSC expansion could be induced only in the basal-like subtype. Alternatively, some genes whose products inhibit CSC expansion may be suppressed by JAG1- or RBPJ-mediated signalling, as it has been reported that JAG1 suppresses the expression of NOTCH target genes by the nuclear translocation of the JAG1 cytoplasmic fragment generated by γ-secretase-dependent processing [44] , and that RBPJ is also involved in the suppression of NOTCH target gene expression [45] . Analyses of clinical data revealed that the NF-κB-JAG1-NOTCH axis-dependent regulation of the CSC population observed in various breast cancer cell lines likely operates in vivo . The NF-κB target genes are highly expressed in basal-like breast tumours when compared with luminal-like and ERBB2-enriched subtypes. Furthermore, JAG1 expression is significantly correlated with the expression of the NF-κB-target genes only in basal-like breast tumours. These results strongly suggest the presence of NF-κB-mediated JAG1 expression in basal-like breast cancer in vivo . More importantly, JAG1 expression levels correlated well with the metastasis-free survival rates of basal-like breast cancer patients, but not with those of patients with other breast cancer subtypes. These results suggest that the intratumoural NF-κB-JAG1-NOTCH axis has a crucial role in regulating the CSC population of basal-like breast tumours. Several groups have recently proposed that basal-like breast cancer originates from the luminal progenitor cell population [16] , [17] , [19] , which exhibits higher NF-κB activation levels when compared with MaSCs and basal myoepithelial cells [46] . Therefore, NF-κB activation in basal-like breast cancer cells and luminal progenitors may be upregulated by similar, not-yet-identified mechanisms in addition to the enhanced NIK expression. Two mechanisms have been reported for NF-κB-dependent JAG1 induction. First, NF-κB directly activates the JAG1 promoter [47] . Second, JAG1 expression is induced by signals activated by IL-6, whose expression is directly induced by NF-κB [48] . Although cell–cell contact-independent effects exist between high-NF-κB cells and CSCs for the regulation of the CSC population, a neutralizing antibody against IL-6 or IL-8 was unable to abrogate the TNFα-induced or IKKβ-mediated expansion of the CSC population. These results strongly suggest that JAG1 is a direct target gene of NF-κB. Therefore, the NF-κB-dependent inducibility of JAG1 may be attributed to the open chromatin structure of the JAG1 locus that is specifically formed in the basal-like subtype. In addition to elucidating the functional link between NF-κB and NOTCH signalling in regulating the CSC population, our study contributes to the development of therapeutic strategies. RANK-mediated NF-κB activation is essential for MaSC proliferation [39] ; therefore, inhibiting NF-κB activation exerts profound effects on normal breast development, which is not significantly affected by the inhibition of NOTCH signalling [26] . In addition, given that GSI treatment significantly inhibits the NF-κB-mediated expansion of the CSC population, specific JAG1 targeting may be a promising approach. Further studies on niches that maintain CSCs must be performed to develop effective therapeutic strategies against basal-like breast cancers. Plasmids and reagents Human cDNAs encoding IκBαSR (S32A/S36A), IKKβ, IKKβEE (S177E/S181E), JAG1, GFP and RFP cDNAs were generated by PCR and inserted into the retroviral vector pMXs, which was obtained from T. Kitamura (University of Tokyo, Japan). The antibodies used were as follows: anti-IKKβ (1:1,000, no. 2684), anti-RELB (1:1,000, no. 4922), anti-NIK (1:1,000, no. 4994), anti-Cleaved NOTCH1 (1:1,000, no. 4147) and anti-RBPJ (1:1,000, no. 5313) (Cell Signalling Technology, Danvers, MA, USA); anti-acetyl-histone H3 (cat. no. 06-599), anti-p52 (1:1,000; cat. no. 05-361) and anti-tubulin (1:2,000; cat. no. CP06) (Millipore, Darmstadt, Germany); anti-Notch1 (1:1,000, sc-32745) (Santa Cruz Biotechnology, Santa Cruz, CA, USA); anti-human CD44-FITC (1:50; no. 560977), anti-human CD44-biotin (1:50; no. 555477), anti-human CD24-PE (1:50; no. 555428) and anti-human CD49f-PE/Cy5 (1:50; no. 551129) (BD Pharmingen, San Diego, CA, USA); anti-human EpCAM-PerPC/Cy5.5 (1:50; no. 324212) (Biolegend, San Diego, CA, USA); a mouse epithelial cell enrichment cocktail (1:20; a mixture of biotinylated antibodies against CD45, TER119 and CD31; STEMCELL Technologies, Vancouver, Canada); anti-mouse CD24-FITC (1:50; eBioscience, San Diego, CA, USA); and anti-TNFα (2 μg ml −1 ; AF-210-NA), anti-IL-6 (2 μg ml −1 ; AF-227-NA) and anti-IL-8 (2 μg ml −1 ; AF-208-NA) (R&D Systems, Minneapolis, MN, USA). The reagents used were as follows: N -[ N -(3,5-difluorophenacetyl)- L -alanyl]- S -phenylglycine t -butyl ester, L685,458 and MG132 (Peptide Institute, Osaka, Japan); epidermal growth factor and basic fibroblast growth factor (BD Pharmingen); TNFα, TGFβ, IL-6 and IL-8 (Sigma-Aldrich, St Louis, MO, USA); 7-amino-actinomycin D (7AAD) (Millipore); streptavidin-ECD (1:10; Beckman Coulter, Fullerton, CA, USA); and slow-release MPA pellets (Innovative Research of America, Sarasota, FL, USA). Cell culture and transfection Human breast cancer cell lines were obtained from the Cell Resource Center for Biomedical Research, Tohoku University (MCF7), and purchased from the American Type Culture Collection (BT-549, HCC1143, HCC1937, HCC1954, HCC38, HCC70, MDA-MB-231, MDA-MB-436, MDA-MB-453, MDA-MB-468 and T-47D). Plat-E and Plat-A retrovirus packaging cells were kindly provided by Dr Kitamura (Institute of Medical Science, University of Tokyo, Tokyo, Japan). All cell lines were cultured according to the recommendations of the supplier. For the retrovirus-mediated gene transfer, the packaging Plat-A and Plat-E cells were transfected with the pMX plasmids by the calcium phosphate method, and virus stocks were prepared by collecting the culture medium. Human basal-like breast cancer cell lines were infected with the virus stock in the presence of 6 μg ml −1 polybrene (Sigma-Aldrich) followed by selection with puromycin; the resultant cell pools were used. EMSA and quantification of NF -κ B activation Cells were collected at 24 h after medium change. Nuclear extracts were prepared, and EMSAs were then performed as described previously [49] . Quantification of relative NF-κB activities in breast cancer cell lines has been described previously [5] . Briefly, intensities of retarded bands corresponding to the NF-κB and DNA complex were measured with a BAS2000 Bioimage analyser (Fuji Film, Tokyo, Japan), and the NF-κB activation level of each cell line was normalized to that of TNFα-stimulated Jurkat cells. Identification of CSCs by flow-cytometry analysis Breast cancer cells were stained with anti-human CD44-FITC, anti-human CD24-PE and anti-human EpCAM-PerPC/Cy5.5 antibodies in the presence of 7AAD (1 μg ml −1 ) in PBS with 1% FBS for 30 min at 4 °C; they were then analysed using an Epics XL flow cytometer (Beckman Coulter, Brea, CA, USA). The CSC and non-CSC populations were sorted on a FACSAria flow cytometer (BD Biosciences, San Jose, CA, USA) after staining as described above. Aldehyde dehydrogenase (ALDH) activity was measured using the ALDEFLUOR kit (STEMCELL Technologies) as previously described [21] . Cells were incubated in ALDEFLUOR assay buffer containing 1 μM ALDH substrate. As a negative control, each cell sample was stained under identical conditions with 15 μM of diethylaminobenzaldehyde, a specific ALDH inhibitor. After 30 min of incubation at 37 °C, the cells were analysed using an Epics XL flow cytometer. In vitro co-culture assay GFP-labelled cell lines with intact NF-κB activation (1 × 10 4 cells) were mixed with an unlabelled corresponding cell line that expresses IKKβ, IκBαSR or Jag1 (1 × 10 5 cells) in six-well plates. Cells were then detached from the plates and stained with anti-human CD44-biotin/streptavidin-ECD (1:10), anti-human CD24-PE (1:50) and anti-human EpCAM-PerPC/Cy5.5 (1:50) antibodies in the presence of 7AAD (1 μg ml −1 ) in PBS with 1% FBS for 30 min at 4 °C; they were then analysed using an Epics XL flow cytometer (Beckman Coulter). GFP + cells were sorted on a FACSAria flow cytometer (BD Biosciences). Sphere-formation assay Breast cancer cells were dissociated into single-cell suspensions by trypsinization. The cells (100 cells per ml in each well) were then seeded into 24-well ultralow-attachment plates (Corning, Corning, NY, USA) in Mammary Epithelial Basal Medium (Lonza, Walkersville, MD, USA) supplemented with 10 ng ml −1 epidermal growth factor, 10 ng ml −1 basic fibroblast growth factor and B27 (Life Technologies). After 7 days, the spheres (>50 μm) were counted to determine the sphere-forming efficiency. Under these conditions, approximately 90% of the mammospheres were derived from a single cell ( Supplementary Fig. S3 ). Tumorigenicity studies Animal research complied with protocols approved by the Committee for Animal Experimentation of the Waseda University. Breast cancer cells were dissociated into single-cell suspensions by trypsinization. The indicated numbers of cells in 100 μl of RPMI1640 (Wako, Tokyo, Japan) containing 50% Matrigel (BD Biosciences) were injected into the fat pads of 7-week-old female NOD/SCID mice (Clea Japan, Kanagawa, Japan). Ten weeks after injection, the mice were euthanised and necropsied, and the formed tumours were counted. Western blotting Whole-cell lysates were separated by SDS–polyacrylamide gel electrophoresis and transferred to polyvinylidene difluoride membranes (Immobilon P; Millipore). The membranes were then incubated with primary antibodies. Immunoreactive proteins were visualized with anti-rabbit or anti-mouse IgG conjugated to horseradish peroxidase (GE Healthcare, Piscataway, NJ, USA), which was followed by processing with an ECL detection system (GE Healthcare). Full-length images of immunoblots are shown in Supplementary Fig. S9 . Quantitative real-time reverse transcriptase PCR assays Total RNA was isolated with the Trizol reagent (Life Technologies). cDNA was synthesized from 1 μg of total RNA with Prime Script II (Takara Bio, Shiga, Japan). Quantitative real-time PCR analysis was performed on a Life Technologies 7300 Fast Real-Time PCR System using FastStart Universal SYBR Green Master Mix (Roche, Basel, Switzerland). The level of β-actin expression was used to normalize the data. The primers used for real-time reverse transcriptase PCR are described in Supplementary Table S1 . Chromatin immunoprecipitation assay A chromatin immunoprecipitation assay was performed as described previously [36] . Anti-acetyl-histone H3 was used for immunoprecipitation. The immunoprecipitation efficiency of the NIK promoter region (−263 to −152) was analysed by real-time PCR using a FastStart Universal SYBR Green Master (Roche) according to the manufacturer’s instructions. The primers used were 5′-ACATCGTCCGGAAATAGTGC-3′ and 5′-CCTACGCCAACCAATGAGAC-3′. Preparation of primary mouse cells The preparation of bone marrow-derived macrophages was performed as described previously [50] . Immortalized mouse mammary fibroblast cells were established from primary mouse mammary fibroblast cells via the retrovirus-mediated expression of SV40 Large T antigens. Cells were cultured in DMEM (Nissui, Tokyo, Japan) supplemented with 10% FBS. For the analysis of Jag1 mRNA expression in primary mammary epithelial cells, slow-release MPA pellets were implanted into 7-week-old female C57/B6J mice (Japan SLC, Hamamatsu, Japan) as previously described [38] . Three weeks after implantation, cells were isolated from the mouse mammary fat pads as previously described and stained with a mouse epithelial cell enrichment cocktail (a mixture of biotinylated antibodies against CD45, TER119 and CD31), streptavidin-ECD, anti-mouse CD24-FITC, anti-human CD49f-PE/Cy5 and 1 μg ml −1 7AAD. The cells were sorted, with the FACSAria Lineage – CD24 high CD49f mid cells as the luminal epithelial cells and the Lineage – CD24 mid CD49f high cells as the basal epithelial cells. Construction of the short hairpin RNA expression vector The target sequence 5′-GGAGCACATTTGCAGTGAATT-3′ was used to silence human JAG1 expression; 5′-GCTGGAAGACAGTACTTTAGA-3′ (shRBPJ no. 1) and 5′-GCACGTTAGGTGGTTAAATCA-3′ (shRBPJ no. 2) were used for human RBPJ expression; 5′-GGTGTGAAAGTCCAAATACAG-3′ (shNIK no. 1) and 5′-GGAGGAATACCTAGTGCATGC-3′ (shNIK no. 2) were used for human NIK expression; and the firefly luciferase-targeted sequence 5′-GATTTCGAGTCGTCTTAATGT-3′ was used as a control. A construct comprising the sense and anti-sense sequences with an intervening 11-bp loop sequence (5′-GTGTGCTGTCC-3′) was inserted between the Bgl II and Hin dIII sites of the pSUPER.retro.puro vector (OligoEngine, Seattle, WA, USA). Clinical analysis A hierarchical clustering analysis of publicly available cDNA microarray data derived from 534 primary mammary tumour samples ( tcga-data.nci.nih.gov/ ; The Cancer Genome Atlas) [31] was performed using the GenePattern software program ( www.broad.mit.edu/cancer/software/genepattern ; Broad Institute, MA, USA) [50] . Each cluster was classified by the marker gene expression of each breast cancer subtype. A GSEA ( www.broadinstitute.org/gsea/index.jsp ; Broad Institute) [33] , [34] and Extraction of Expression Module analysis [35] were performed for each breast cancer subtype with the NF-κB-dependent gene set ‘TIAN_TNF_SIGNALING_VIA_NFKB’ ( www.broadinstitute.org/gsea/msigdb/cards/TIAN_TNF_SIGNALING_VIA_NFKB.html ; Broad Institute) [32] . Statistics Statistically significant differences between the mean values were determined using a two-tailed Student’s t -test and Fisher’s exact test. All data are representative of three independent experiments. The values represent the means of triplicate samples±s.d. P -values <0.05 were considered statistically significant. How to cite this article: Yamamoto, M. et al . NF-κB non-cell-autonomously regulates cancer stem cell populations in the basal-like breast cancer subtype. Nat. Commun. 4:2299 doi: 10.1038/ncomms3299 (2013).